Haematopoietic focal adhesion kinase deficiency alters haematopoietic homeostasis to drive tumour metastasis Metastasis is the main cause of cancer-related death and thus understanding the molecular and cellular mechanisms underlying this process is critical. Here, our data demonstrate, contrary to established dogma, that loss of haematopoietic-derived focal adhesion kinase (FAK) is sufficient to enhance tumour metastasis. Using both experimental and spontaneous metastasis models, we show that genetic ablation of haematopoietic FAK does not affect primary tumour growth but enhances the incidence of metastasis significantly. At a molecular level, haematopoietic FAK deletion results in an increase in PU-1 levels and decrease in GATA-1 levels causing a shift of hematopoietic homeostasis towards a myeloid commitment. The subsequent increase in circulating granulocyte number, with an increase in serum CXCL12 and granulocyte CXCR4 levels, was required for augmented metastasis in mice lacking haematopoietic FAK. Overall our findings provide a mechanism by which haematopoietic FAK controls cancer metastasis. Understanding the molecular and cellular basis of metastasis still remains a major challenge in current cancer research. Focal adhesion kinase (FAK) is a cytoplasmic protein-tyrosine kinase that localizes mainly at focal adhesion sites, and is one of the central players in integrin and growth factor receptor mediated signalling [1] , [2] . FAK also has important non-kinase functions [3] . FAK is overexpressed in many human cancer cells and has thus emerged as an anticancer target [4] , [5] , [6] , [7] , [8] . This has led to the development of FAK inhibitors although off-target effects are apparent [9] , [10] , [11] . Moreover, evidence suggests that FAK may have pleiotropic effects and some work has pointed to FAK being a negative regulator of metastasis. For example, a study of cervical cancer has shown that even though FAK expression was found to be upregulated in tumour cells when compared with normal cervical epithelium, weak FAK expression was significantly correlated with poor overall survival [12] . In addition, Zheng et al. [13] have suggested that FAK-dephosphorylation in tumour cells is important for Ras-mediated metastasis. These data suggest that FAK may not be required for metastasis and that the precise role for FAK in metastasis may be more complex than initially thought. They also raise the question of the importance of stromal FAK in the metastatic process. The tumour stromal compartment has been shown to have an important role in metastasis [14] , [15] , [16] . Within the tumour stroma, bone marrow-derived cells, specifically myeloid, have been identified as regulators of tumour invasiveness and implicated in organ-specific tumour metastasis [17] , [18] . A heterogeneous population of cells that comprises myeloid progenitor cells and immature myeloid cells, also named myeloid-derived suppressor cells (MDSCs), has been correlated with clinical stage and metastatic burden [19] , [20] . MDSCs are a mixture of myeloid cells with characteristics of monocytes and granulocytes and are generally described by the co-expression of the mouse markers CD11b and Gr1 (CD11b + Gr1 + ) [21] , [22] . Their expansion at metastatic sites generates an immunosuppressive niche that suppresses T cell activation, proliferation and cytotoxicity and also suppresses NK cell cytotoxicity [23] , [24] , [25] , [26] . These cells have been shown to facilitate tumour cell seeding and colonization at metastatic sites and are thereby thought to drive metastasis [27] , [28] , [29] . In short, analysis of tumour cells has suggested that FAK is required for tumour metastasis, but the role of stromal or haematopoietic-derived FAK in this process is poorly understood. We have tested the requirement of haematopoietic FAK in metastasis using genetic ablation approaches in combination with haematopoietic transplant experiments. Here we establish that decreased expression of FAK in the haematopoietic compartment generates a pro-metastatic microenvironment that actually enhances tumour cell colonization and metastasis. Our data highlight a role for haematopoietic FAK as a negative, rather than positive, regulator of tumour cell metastasis via the control of haematopoietic homeostasis and mobilization of CD11b + Gr1 + cells. FAK deletion increases metastases in the RIP-Tag2 model A genetic approach was used to ablate FAK globally to study the effect of FAK deletion on tumour metastasis. We generated a tamoxifen-inducible model for FAK deletion in adult mice, RERTn ERT/ERT Cre;FAK fl/fl and confirm efficient FAK deletion at the protein level in this system ( Supplementary Figs 1A–D, 2A, B ) [30] , [31] , [32] . RERTn ERT/ERT Cre mice have been used previously to induce global deletion of target genes [31] . Non-induced RERTn ERT/ERT Cre;FAK fl/fl mice were viable and fertile with no obvious defects. The effect of FAK deletion on metastasis was first analysed in RIP-Tag2 mice, a well-studied, spontaneous model of pancreatic cancer that expresses the SV40 T antigen (Tag) under the control of the rat insulin promoter [33] . Expression of Tag in pancreatic islet β-cells leads to the development of hyperplastic lesions at 6–8 weeks of age of which a fraction will progress into highly vascularized β-cell tumours at 10–14 weeks of age. These tumours have been reported to invade and spread to lymph nodes and liver [34] . RIP-Tag2 mice die by 16 weeks of age [33] . RIP-Tag2 mice were crossed with RERTn ERT/ERT Cre;FAK fl/fl (RERTFAK KO ) or control FAK fl/fl (RERTFAK WT ) mice generating RIP-Tag2;RERTFAK KO and RIP-Tag2;RERTFAK WT mice respectively. Mice were treated with tamoxifen from 9 weeks of age to induce FAK deletion in both tumour and stromal compartments. Total pancreatic tumour burden was not statistically different between genotypes at 15 weeks of age ( Fig. 1a ). Pancreatic tumours in RIP-Tag2 mice are classified into three levels of progression: encapsulated, the least aggressive form; invasive type I, where the invasive front of the tumour begins to penetrate into the surrounding pancreas; and invasive type II, where the invasive front of the tumour engulfs islands of normal pancreas [34] , [35] . Quantification of Tag-positive pancreas sections revealed that FAK deletion had no significant effect on tumour invasiveness ( Fig. 1b ). Histological analysis of metastases to the peri-pancreatic lymph nodes also showed no statistically significant differences between genotypes in incidence of metastasis or percentage of lymph nodes with metastases ( Supplementary Fig. 3A ). In contrast the incidence of metastases and number of metastases per liver were significantly higher in RIP-Tag2;RERTFAK KO when compared with RIP-Tag2;RERTFAK WT mice ( Fig. 1c–e ). These data show that when FAK is deleted globally, RIP-Tag2 primary tumour burden is not affected but metastasis is enhanced. 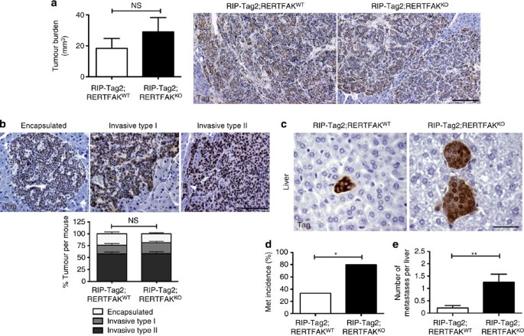Figure 1: FAK deficiency enhances metastasis in theRIP-Tag2model. RIP-Tag2;RERTFAKWTand RIP-Tag2;RERTFAKKOmice started tamoxifen treatment at 9 weeks of age and were necropsied at 15 weeks of age. Histological analysis was performed in five different depth areas 100 μm apart of pancreas and liver with immunohistochemical staining for the tumour marker SV40 T antigen (Tag). (a) Primary tumour burden in RIP-Tag2;RERTFAKWTand RIP-Tag2;RERTFAKKOmice. Bar chart represents the total macroscopic tumour burden+s.e.m.,n=10–13 mice per genotype. Representative images of Tag immunostained sections primary tumours are shown. NS, not statistically significant, Student’st-test. (b) Histological images of Tag immunostained tumour sections at different stages of invasiveness are shown. Quantification of tumour invasiveness is presented as the percentage of encapsulated islet tumours (encapsulated), microinvasive carcinomas (invasive type I), and fully invasive carcinomas (invasive type II) in RIP-Tag2;RERTFAKWTand RIP-Tag2;RERTFAKKOmice. NS, not statistically significant, Mann–Whitney test. (c) Representative images of Tag-positive liver metastases. Bar charts represent (d) incidence of metastasis to the liver or (e) number of metastases per liver. Scale bars, (a) 500 μm, (b) 200 μm, (c)50 μm. *P<0.05; **P<0.01; Mann–Whitney test. Figure 1: FAK deficiency enhances metastasis in the RIP-Tag2 model. RIP-Tag2;RERTFAK WT and RIP-Tag2;RERTFAK KO mice started tamoxifen treatment at 9 weeks of age and were necropsied at 15 weeks of age. Histological analysis was performed in five different depth areas 100 μm apart of pancreas and liver with immunohistochemical staining for the tumour marker SV40 T antigen (Tag). ( a ) Primary tumour burden in RIP-Tag2;RERTFAK WT and RIP-Tag2;RERTFAK KO mice. Bar chart represents the total macroscopic tumour burden+s.e.m., n =10–13 mice per genotype. Representative images of Tag immunostained sections primary tumours are shown. NS, not statistically significant, Student’s t -test. ( b ) Histological images of Tag immunostained tumour sections at different stages of invasiveness are shown. Quantification of tumour invasiveness is presented as the percentage of encapsulated islet tumours (encapsulated), microinvasive carcinomas (invasive type I), and fully invasive carcinomas (invasive type II) in RIP-Tag2;RERTFAK WT and RIP-Tag2;RERTFAK KO mice. NS, not statistically significant, Mann–Whitney test. ( c ) Representative images of Tag-positive liver metastases. Bar charts represent ( d ) incidence of metastasis to the liver or ( e ) number of metastases per liver. Scale bars, ( a ) 500 μm, ( b ) 200 μm, ( c )50 μm. * P <0.05; ** P <0.01; Mann–Whitney test. Full size image Stromal FAK deficiency increases experimental metastasis Tumour growth and metastasis is regulated not only by the tumour cells themselves but also by the host or stromal compartment. To dissect the role of FAK within the host or stromal compartment from that in the tumour compartment, an experimental metastasis approach was employed. Syngeneic mouse B16 melanoma cells, which express FAK, were injected via the tail vein into RERTFAK KO and RERTFAK WT mice. At 19 days post B16 cell injection, significantly elevated numbers of metastatic nodules were observed in several organs including the lungs, liver and bones of RERTFAK KO mice when compared with controls ( Fig. 2a ). Sections of tissues were stained with haematoxylin and eosin and metastases counted. Results showed a significant increase in the total number of metastases in RERTFAK KO mice when compared with controls ( Fig. 2b–d ). These data indicate that loss of FAK in the stromal compartment is sufficient to increase experimental B16 tumour metastasis. 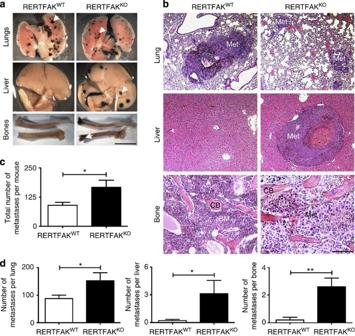Figure 2: Loss of stromal FAK increases experimental metastasis. RERTFAKWTand RERTFAKKOmice were injected via the tail vein with B16 mouse melanoma tumour cells and analysed 19 days post inoculation. Metastases in lungs, liver and bones of RERTFAKWTand RERTFAKKOmice: (a) Macroscopic images and (b) representative images of haematoxylin and eosin stained sections. (c) Bar chart represents the mean number of metastases per mouse+s.e.m. (d) Bar charts show mean number of metastases to the lung, liver or bone+s.e.m.,n=10–12 mice per genotype. BM, bone marrow; CB, calcified bone; Met, metastases; white arrow, metastases. Scale bars, (a) 1 cm; (b) 200 μm. *P<0.05; **P<0.01, Mann–Whitney test. Figure 2: Loss of stromal FAK increases experimental metastasis. RERTFAK WT and RERTFAK KO mice were injected via the tail vein with B16 mouse melanoma tumour cells and analysed 19 days post inoculation. Metastases in lungs, liver and bones of RERTFAK WT and RERTFAK KO mice: ( a ) Macroscopic images and ( b ) representative images of haematoxylin and eosin stained sections. ( c ) Bar chart represents the mean number of metastases per mouse+s.e.m. ( d ) Bar charts show mean number of metastases to the lung, liver or bone+s.e.m., n =10–12 mice per genotype. BM, bone marrow; CB, calcified bone; Met, metastases; white arrow, metastases. Scale bars, ( a ) 1 cm; ( b ) 200 μm. * P <0.05; ** P <0.01, Mann–Whitney test. Full size image Haematopoietic FAK deletion increases RIP-Tag2 metastases Tumour cell survival in the circulation, seeding at distant sites, invasion and dissemination are all processes dependent on the tumour microenvironment. These processes have been shown to involve many cell types but the molecular mechanisms underlying the role of bone marrow-derived cells is still unclear [18] , [36] . To dissect the requirement of FAK within the haematopoietic compartment from that in the whole stromal compartment, we undertook an adoptive transfer approach. Briefly, lethally irradiated 6-week-old female RIP-Tag2 mice were transplanted with bone marrow from either male RERTn ERT/ERT Cre;FAK fl/fl or control FAK fl/fl cre negative mice generating RIP-Tag2;BMFAK KO and RIP-Tag2;BMFAK WT chimeras, respectively. Two weeks after bone marrow transplantation, mice were treated with tamoxifen to induce FAK deletion predominantly in the haematopoietic compartment. At 16 weeks of age, necropsies were performed and showed that RIP-Tag2;BMFAK KO mice had no significant difference in pancreatic tumour burden when compared with RIP-Tag2;BMFAK WT controls ( Fig. 3a ). It is noteworthy that tumour burden in both genotypes was lower than predicted for RIP-Tag2 mice at this age most likely because the animals were irradiated, as reported previously [37] . Quantification of Tag immunostained pancreas sections revealed that haematopoietic FAK deletion had no significant effect on tumour invasiveness ( Fig. 3b ) suggesting that haematopoietic FAK is not sufficient to modulate primary tumour growth or invasion per se . Histological analysis of metastases to the peri-pancreatic lymph nodes showed very low numbers of lymph node metastases in both genotypes and no statistically significant differences between them ( Supplementary Fig. 3B ). Despite this, the incidence of liver metastasis was significantly higher in RIP-Tag2;BMFAK KO when compared with RIP-Tag2;BMFAK WT mice ( Fig. 3c,d ). Unexpectedly, RIP-Tag2;BMFAK KO mice also presented an increased incidence of lung metastases, an organ that has not been previously reported to display RIP-Tag2 metastasis ( Fig. 3c,d ). The overall incidence of metastasis was statistically increased in RIP-Tag2;BMFAK KO mice when compared with RIP-Tag2;BMFAK WT controls ( Fig. 3d ). These data from a spontaneous model of cancer show that deficiency of haematopoietic FAK is sufficient to enhance tumour metastasis. 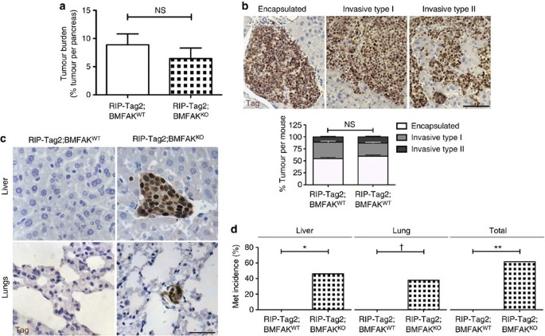Figure 3: Haematopoietic FAK deficiency enhancesRIP-Tag2metastases. RIP-Tag2mice were transplanted at 6 weeks of age, and tamoxifen treated 2–3 weeks thereafter generating RIP-Tag2;BMFAKWTand RIP-Tag2;BMFAKKOchimeras. Mice were necropsied at 16 weeks of age. Histological analysis was performed in six different depth areas 100 μm apart of pancreas, liver and lungs with immunohistochemical staining for the tumour marker SV40 T antigen (Tag). (a) Tumour burden in RIP-Tag2;BMFAKWTand RIP-Tag2;BMFAKKOmice. Bar chart represents the proportion of tumour burden as a % of tumour area per animal normalized to total pancreas area+s.e.m.,n=7–13 mice per genotype. NS, not statistically significant, Mann–Whitney test. (b) Quantification of tumour invasiveness is presented as the percentage of encapsulated islet tumours (encapsulated), microinvasive carcinomas (invasive type I), and fully invasive carcinomas (invasive type II) in RIP-Tag2;BMFAKWTand RIP-Tag2;BMFAKKOmice. NS, not statistically significant, Mann–Whitney test. Scale bar, 200 μm. (c) Representative images of Tag immunostained sections of liver and lung. Metastases to liver and lungs are shown. Scale bar, 50 μm. (d) Bar charts represent incidence of metastasis to either liver or lung or total percentage of animals with metastases.†P<0.058; *P<0.05; **P<0.01, Mann–Whitney test. Figure 3: Haematopoietic FAK deficiency enhances RIP-Tag2 metastases. RIP-Tag2 mice were transplanted at 6 weeks of age, and tamoxifen treated 2–3 weeks thereafter generating RIP-Tag2;BMFAK WT and RIP-Tag2;BMFAK KO chimeras. Mice were necropsied at 16 weeks of age. Histological analysis was performed in six different depth areas 100 μm apart of pancreas, liver and lungs with immunohistochemical staining for the tumour marker SV40 T antigen (Tag). ( a ) Tumour burden in RIP-Tag2;BMFAK WT and RIP-Tag2;BMFAK KO mice. Bar chart represents the proportion of tumour burden as a % of tumour area per animal normalized to total pancreas area+s.e.m., n =7–13 mice per genotype. NS, not statistically significant, Mann–Whitney test. ( b ) Quantification of tumour invasiveness is presented as the percentage of encapsulated islet tumours (encapsulated), microinvasive carcinomas (invasive type I), and fully invasive carcinomas (invasive type II) in RIP-Tag2;BMFAK WT and RIP-Tag2;BMFAK KO mice. NS, not statistically significant, Mann–Whitney test. Scale bar, 200 μm. ( c ) Representative images of Tag immunostained sections of liver and lung. Metastases to liver and lungs are shown. Scale bar, 50 μm. ( d ) Bar charts represent incidence of metastasis to either liver or lung or total percentage of animals with metastases. † P <0.058; * P <0.05; ** P <0.01, Mann–Whitney test. Full size image Haematopoietic FAK deletion increases B16 metastases We next tested the effect of haematopoietic FAK deficiency on experimental tumour metastasis by injecting B16 mouse melanoma tumour cells in the tail vein of BMFAK WT and BMFAK KO mice. Results showed that deficiency of FAK in the haematopoietic compartment alone was sufficient to increase the number of tumour metastases in BMFAK KO mice significantly when compared with controls ( Fig. 4a ). The presence of this increased number of metastases was confirmed by histological analysis of the lungs, liver and bones from BMFAK KO mice and respective controls ( Fig. 4b ). Quantification revealed a significant increase in the number of B16 nodules not only in BMFAK KO lungs, but also in the livers and bones of these mice when compared with controls ( Fig. 4c,d ). Validation of the adoptive transfer approach is given in Supplementary Figs 2C and 4 . Together, these data indicate that the loss of stromal FAK, solely within the haematopoietic compartment, is sufficient to control tumour metastasis. 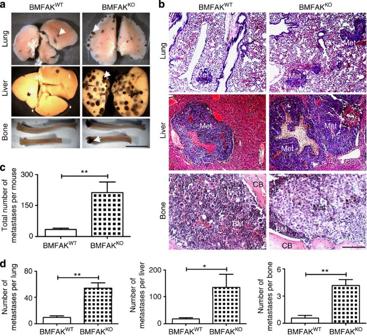Figure 4: Haematopoietic FAK deletion increases B16 metastasis. BMFAKWTand BMFAKKOmice were injected with B16 mouse melanoma tumour cells via the tail vein in experimental metastasis experiments and analysed 15–17 days post tumour cell injection. Metastases in lungs, liver and bones from BMFAKWTand BMFAKKOmice: (a) Macroscopic images and (b) representative images of haematoxylin and eosin stained sections. (c) Bar chart shows mean number of metastases per mouse,+s.e.m. (d) Bar charts show mean number of metastases to the lung, liver and bone+s.e.m.,n=9 mice per genotype. BM, bone marrow; CB, calcified bone; Met, metastases; white arrow, metastases. Scale bars, (a) 1 cm; (b) 200 μm. *P<0.05; **P<0.01, Mann–Whitney test. Figure 4: Haematopoietic FAK deletion increases B16 metastasis. BMFAK WT and BMFAK KO mice were injected with B16 mouse melanoma tumour cells via the tail vein in experimental metastasis experiments and analysed 15–17 days post tumour cell injection. Metastases in lungs, liver and bones from BMFAK WT and BMFAK KO mice: ( a ) Macroscopic images and ( b ) representative images of haematoxylin and eosin stained sections. ( c ) Bar chart shows mean number of metastases per mouse,+s.e.m. ( d ) Bar charts show mean number of metastases to the lung, liver and bone+s.e.m., n =9 mice per genotype. BM, bone marrow; CB, calcified bone; Met, metastases; white arrow, metastases. Scale bars, ( a ) 1 cm; ( b ) 200 μm. * P <0.05; ** P <0.01, Mann–Whitney test. Full size image A recent paper by Catena et al. [38] showed that expression of thrombospondin—1 (Tsp-1) by Cd11b + Gr1 + cells generates a metastatic refractory microenvironment. In line with this study we have observed lower levels of Tsp-1 in bone marrow from RERTFAK KO animals that show increased numbers of metastases ( Supplementary Figs 5A and 6A ). In the same study, tumours cells that secrete prosaposin (Psap) induce Tsp-1 expression in CD11b + Gr1 + cells causing them to behave as metastasis refractory cells [38] . To assess the relevance of prosaposin in our system, we first analysed prosaposin levels in B16F0 and B16F10 tumour cells used in our study. Both B16F0 and B16F10 showed no detectable levels of prosaposin and we saw no effect of introducing prosaposin in the phenotypes observed in BMFAK KO mice; thus we conclude that, for the purposes of our experiments, prosaposin is unlikely to be involved ( Supplementary Figs 5B–D and 6B–C ). FAK deficiency shifts HSCs towards a myeloid commitment Our results suggest that metastasis is enhanced in mice lacking haematopoietic FAK. It is conceivable that loss of FAK could be compensated for by the upregulation of other functionally related molecules. Pyk2 is a member of the FAK family of tyrosine kinases and has been shown to compensate for FAK loss in previous studies [39] , [40] , [41] . Western blot analysis of haematopoietic lysates from RERTFAK KO and RERTFAK WT mice showed no significant changes in the levels of Pyk2 between genotypes ( Supplementary Fig. 7 ). In addition the expression levels of other focal contact proteins such as paxillin, vinculin and talin were also unchanged between RERTFAK KO and RERTFAK WT samples ( Supplementary Figs 2D and 7 ). These data suggest that at least these candidate genes were unlikely to be compensating for the loss of FAK. To understand the mechanism that drives the increased metastasis in the absence of FAK we sought to phenotypically characterize the haematopoietic compartment of RERTFAK WT and RERTFAK KO mice. The role of bone marrow-derived cells in tumour progression and metastasis has been studied extensively, but the role of FAK in this process is not known [18] , [29] , [36] . Recent evidence has suggested that FAK can regulate haematopoietic homeostasis in the bone marrow [42] . Using flow cytometric analysis we have characterized haematopoietic stem cells (HSCs) and committed progenitors in bone marrow from RERTFAK WT and RERTFAK KO mice ( Fig. 5a ). We observed an increase in phenotypically defined long-term repopulating stem cells LT-HSCs (Lin low c-kit + Sca-1 + CD34 − Flk-2 − ) in RERTFAK KO mice when compared with RERTFAK WT control mice with only a tendency for an increase in short-term repopulating stem cells ST-HSCs (Lin low c-kit + Sca-1 + CD34 + Flk-2 − ; Fig. 5b,c ). No differences were observed in multipotent progenitors MPP (Lin low c-kit + Sca-1 + CD34 + Flk-2 + ; Supplementary Fig. 8A ). Analysis of bone marrow-committed progenitors shows an increase in common myeloid progenitor CMP (Lin low c-kit + Sca-1 − CD34 + CD16/32 mid ) in RERTFAK KO when compared with RERTFAK WT mice ( Fig. 5d ). No differences in other bone marrow-committed progenitors, such as common lymphoid progenitor CLP (Lin low c-kit mid Sca-1 mid CD127 + ), granulocyte-monocyte progenitor GMP (Lin low c-kit + Sca-1 − CD34 + CD16/32 bright ) or megakaryocyte and erythroid progenitors MEP (Lin low c-kit + Sca-1 − CD34 + CD16/32 low ) were observed between genotypes ( Supplementary Fig. 8B–D ) [43] . These data suggest that FAK-deficient HSCs are predisposed to a myeloid commitment. To test this hypothesis, we sorted HSCs (Lin low c-kit + Sca-1 + ) from the bone marrow of RERTFAK WT and RERTFAK KO mice and analysed transcription factors involved in myeloid commitment by real time PCR. PU.1 is a transcription factor critically responsible for the activation of myeloid-specific promoters, such as murine neutrophil elastase, granulocyte colony stimulating factor (G-CSF), macrophage (M)-CSF and GM-CSF promoters [44] , [45] . On the other hand, GATA-1 expression has been shown to suppress the myeloid expression program [46] , [47] . FAK KO HSCs had increased PU.1 and decreased GATA-1 expression, when compared with controls. ( Fig. 5e–g ). Together these data show that FAK deletion shifts HSC transcriptional programme towards myeloid lineage commitment. 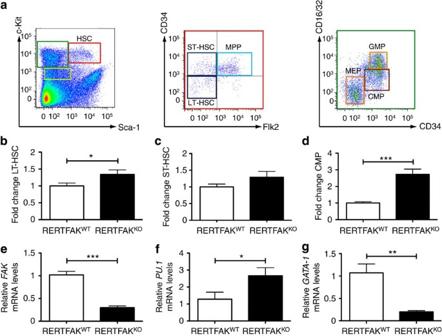Figure 5: FAK deficiency shifts HSCs towards a myeloid commitment. Single-cell suspensions of bone marrow from RERTFAKWTand RERTFAKKOmice were analysed by flow cytometry. (a) Long-term bone marrow-derived haematopoietic stem cells, LT-HSC (Linlowc-kit+Sca-1+CD34−Flk-2−), short-term bone marrow-derived haematopoietic stem cells, ST-HSC (Linlowc-kit+Sca-1+CD34+Flk-2−) and common myeloid progenitors, CMP (Linlowc-kit+Sca-1−CD34+CD16/32mid) in the BM of RERTFAKWTand RERTFAKKOmice were compared. Representative dot blots are shown. Bar charts show fold change of bone marrow LT-HSC (b) ST-HSC (c) and CMP (d)+s.e.m.,n=10–13 mice per genotype. (e–g) HSCs (Linlowc-kit+Sca-1+) were sorted from the bone marrow of RERTFAKWTand RERTFAKKOmice, RNA extracted and reversed transcribed into cDNA. Bar charts show mean (e)FAK, (f)PU.1and (g)GATA-1mRNA levels+s.e.m. quantified by real time PCR,n=3–4 mice/genotype. *P<0.05; **P<0.01; ***P<0.001, Student’st-test. Figure 5: FAK deficiency shifts HSCs towards a myeloid commitment. Single-cell suspensions of bone marrow from RERTFAK WT and RERTFAK KO mice were analysed by flow cytometry. ( a ) Long-term bone marrow-derived haematopoietic stem cells, LT-HSC (Lin low c-kit + Sca-1 + CD34 − Flk-2 − ), short-term bone marrow-derived haematopoietic stem cells, ST-HSC (Lin low c-kit + Sca-1 + CD34 + Flk-2 − ) and common myeloid progenitors, CMP (Lin low c-kit + Sca-1 − CD34 + CD16/32 mid ) in the BM of RERTFAK WT and RERTFAK KO mice were compared. Representative dot blots are shown. Bar charts show fold change of bone marrow LT-HSC ( b ) ST-HSC ( c ) and CMP ( d )+s.e.m., n =10–13 mice per genotype. ( e – g ) HSCs (Lin low c-kit + Sca-1 + ) were sorted from the bone marrow of RERTFAK WT and RERTFAK KO mice, RNA extracted and reversed transcribed into cDNA. Bar charts show mean ( e ) FAK , ( f ) PU.1 and ( g ) GATA-1 mRNA levels+s.e.m. quantified by real time PCR, n =3–4 mice/genotype. * P <0.05; ** P <0.01; *** P <0.001, Student’s t -test. Full size image Loss of BM FAK induces a pro-metastatic microenvironment Granulocytes or polymorphonuclear cells (CD11b + Gr1 hi Ly6C lo+int —PMN) have a short half-life, are quickly mobilized into the circulation and are considered the best indicator of changes in haematopoietic homeostasis [48] , [49] . The increase in common myeloid progenitor was reflected in the periphery by elevated numbers of PMN cells in the blood and spleen of RERTFAK KO mice in the steady state and at various stages after tail vein injection of tumour cells. Increased numbers of granulocytes were observed in the blood ( Fig. 6a ) and spleen ( Fig. 6b ) of unchallenged RERTFAK KO mice, 2–5 h after tumour cell injection (time for tumour cell homing), 24 h after tumour cell injection (time for tumour cell colonization) and at the experimental end point (time of tumour cell establishment). We also observed similar changes in the monocytic fraction of CD11b + Gr1 + cells (CD11b + Gr1 lo+int Ly6C hi —Mon) but to a lesser extent ( Supplementary Fig. 8E–G ). Our data establish that loss of haematopoietic FAK alters haematopoietic homeostasis and increases CD11b + Gr1 + cell mobilization and numbers into the circulation. 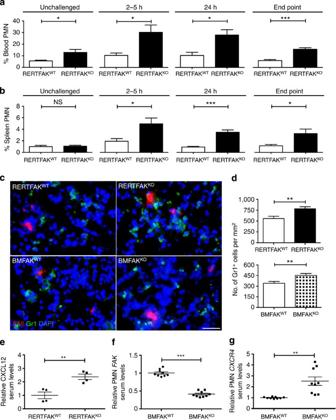Figure 6: Stromal FAK deficiency induces PMN changes. Single-cell suspensions of (a) blood and (b) spleen from RERTFAKWTand RERTFAKKOmice that were either unchallenged or 2–5 h, 24 h and 15 days post tumour cell injection via the tail vein were analysed by flow cytometry. Bar charts show numbers of CD45+CD11b+Gr1hiLy6Clo(PMN) in blood and spleen from RERTFAKWTand RERTFAKKOmice.n=3–4 mice per genotype. (c,d) B16 tumour cells, previously labelled with red cell tracker CMTPX, were injected via the tail vein into RERTFAKWT, RERTFAKKO, BMFAKWTand BMFAKKOmice. Then 2–5 h post injection, lungs were processed and sections immunostained for Gr1+cells. (c) Representative images of B16 tumour cells (red) and Gr1+ cells (green) in RERTFAKWT, RERTFAKKO, BMFAKWTand BMFAKKOlung sections 2–5 h after tumour cell injection. (d) Gr1+cell infiltration into the lungs in RERTFAKWT, RERTFAKKO, BMFAKWTand BMFAKKOmice. Bar charts represent number of Gr1+cell per mm2of lung section+s.e.m.,n=4–5 mice per genotype. (e) Serum levels of CXCL12 in RERTFAKWTand RERTFAKKOmice 24 h after tumour cell injection. Bar chart represents fold change relative to RERTFAKWT+s.e.m. (f,g) CD45+CD11b+Gr1hiLy6Clo(PMN) cells were sorted from the lung of BMFAKWTand BMFAKKOmice 24 h after tumour cell injection, RNA extracted and reversed transcribed into cDNA. Bar charts show meanFAK(f) andCXCR4(g) mRNA levels+s.e.m. quantified by real time PCR,n=8–10 mice per genotype. Scale bar, 100 μm. NS, not statistically significant; *P<0.05; **P<0.01; ***P<0.001, Student’st-test. Figure 6: Stromal FAK deficiency induces PMN changes. Single-cell suspensions of ( a ) blood and ( b ) spleen from RERTFAK WT and RERTFAK KO mice that were either unchallenged or 2–5 h, 24 h and 15 days post tumour cell injection via the tail vein were analysed by flow cytometry. Bar charts show numbers of CD45 + CD11b + Gr1 hi Ly6C lo (PMN) in blood and spleen from RERTFAK WT and RERTFAK KO mice. n =3–4 mice per genotype. ( c , d ) B16 tumour cells, previously labelled with red cell tracker CMTPX, were injected via the tail vein into RERTFAK WT , RERTFAK KO , BMFAK WT and BMFAK KO mice. Then 2–5 h post injection, lungs were processed and sections immunostained for Gr1 + cells. ( c ) Representative images of B16 tumour cells (red) and Gr1+ cells (green) in RERTFAK WT , RERTFAK KO , BMFAK WT and BMFAK KO lung sections 2–5 h after tumour cell injection. ( d ) Gr1 + cell infiltration into the lungs in RERTFAK WT , RERTFAK KO , BMFAK WT and BMFAK KO mice. Bar charts represent number of Gr1 + cell per mm 2 of lung section+s.e.m., n =4–5 mice per genotype. ( e ) Serum levels of CXCL12 in RERTFAK WT and RERTFAK KO mice 24 h after tumour cell injection. Bar chart represents fold change relative to RERTFAK WT +s.e.m. ( f , g ) CD45 + CD11b + Gr1 hi Ly6C lo (PMN) cells were sorted from the lung of BMFAK WT and BMFAK KO mice 24 h after tumour cell injection, RNA extracted and reversed transcribed into cDNA. Bar charts show mean FAK ( f ) and CXCR4 ( g ) mRNA levels+s.e.m. quantified by real time PCR, n =8–10 mice per genotype. Scale bar, 100 μm. NS, not statistically significant; * P <0.05; ** P <0.01; ***P<0.001, Student’s t -test. Full size image Given the increased mobilization and expansion of the CD11b + Gr1 + cells in the blood and spleen at early time points after tumour cell injection, we next analysed whether an increase of these cells was observed at metastatic sites such as the lung. Immunofluorescence for Gr1 showed increased numbers of Gr1 + cells in the lungs of RERTFAK KO and BMFAK KO mice, 2–5 h post tumour cell injection, when compared with RERTFAK WT and BMFAK WT controls, respectively ( Fig. 6c,d ). An increased number of Gr1 + cells has been correlated previously with enhanced metastasis [27] , [28] , [29] . In parallel we noted a decrease in infiltration of CD4 + and CD8 + T cells at early time points after tumour cell injection ( Supplementary Fig. 9A–D ), but no differences in NK cell infiltrate in the lungs of RERTFAK KO or BMFAK KO mice when compared with controls ( Supplementary Fig. 9E, F ). Since no changes in CLP were observed in the bone marrow ( Supplementary Fig. 8B ), it is possible that these T cell changes are a consequence of the increased Gr1 + cell numbers as the latter have been shown previously to have immune suppressive properties [23] , [24] . Metastasis and neutrophil recruitment are dependent on complex cytokine networks. Analysis of serum cytokine levels after tumour cell injection by protein cytokine arrays showed increased levels of CXCL12 in the serum of RERTFAK KO mice ( Fig. 6e ). This coincided with a significant increase in CXCR4 mRNA levels in FAK KO PMNs recruited to the lung after tumour cell injection ( Fig. 6f,g ). CXCL12-CXCR4 axis is involved in metastasis and neutrophil homing [25] , [50] , [51] . The higher levels of CXCR4 expression in FAK KO PMN cells suggest that these cells may have increased propensity to respond to pro-metastatic cytokines such as CXCL12 and home to sites of metastasis. In addition, other inflammatory cytokines such as the complement component C5/C5a was found increased in the serum of RERTFAK KO mice ( Supplementary Fig. 9G ). C5/C5a has previously been shown to be involved in neutrophil recruitment and lung inflammation preceding lung metastasis [52] , [53] . Taken together these data suggest RERTFAK KO mice present a microenvironment that favours the recruitment of PMN to metastatic sites. Gr1 cells govern tumour cell colonization in RERTFAK KO mice FAK deficiency in the haematopoietic compartment resulted in changes in the inflammatory microenvironment that facilitated recruitment of PMN to metastatic sites at early time points after tumour cell injection. To test whether these changes could have an impact on tumour cell homing or colonization, key steps in metastasis, red cell tracker-labelled tumour cells were injected into the tail vein of RERTFAK WT , RERTFAK KO , BMFAK WT and BMFAK KO mice and lungs harvested 2–5 h (to test for homing) and 48 h (to test for colonization) thereafter. Although there were no differences in the numbers of tumour cells homing in the lungs 2–5 h post injection, a significant increase in tumour cell colonization at 48 h post injection was observed in RERTFAK KO and BMFAK KO mice when compared with RERTFAK WT and BMFAK WT controls ( Fig. 7a,b ). Analysis of Ki67 showed that the majority of cells were not proliferating at 48 h post injection and there were no differences between RERTFAK WT and RERTFAK KO mice, suggesting FAK deletion affected the seeding of tumour cells rather than proliferation ( Supplementary Fig. 10A ). 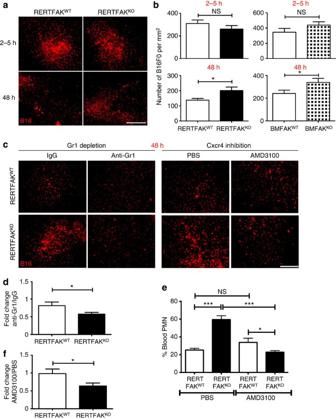Figure 7: Gr1 cells govern tumour cell colonization in RERTFAKKOmice. B16 tumour cells, previously labelled with red cell tracker CMTPX, were injected via the tail vein into RERTFAKWT, RERTFAKKO, BMFAKWTand BMFAKKOmice. (a) Lungs were harvested 2–5 h and 48 h after tumour cell injection to measure the numbers of tumour cells homing and colonizing in the lungs, respectively. Representative stereomicroscopic images of lung surfaces from RERTFAKWTand RERTFAKKOmice are given. (b) Bar charts represent mean number of B16 cells mm−2lung section+s.e.m.,n=5 mice per genotype. (c) Gr1 antibody-depletion of Gr1+ cells or CXCR4 inhibition with AMD3100 in RERTFAKWTand RERTFAKKOmice. Nonspecific IgG or PBS were used as a control. Mice were then injected with red cell tracker CMTPX labelled B16 cells. Representative stereomicroscope images of fresh lungs from both genotypes are given. (d) Bar chart shows fold change relative to IgG of mean number of B16 cells per lung area.n=10–12 mice per test. (e) Single-cell suspensions of blood from RERTFAKWTand RERTFAKKOmice 2 h post tumour cell injection via the tail vein were analysed by flow cytometry. Bar charts show numbers of CD45+CD11b+Gr1hiLy6Clo(PMN) in blood.n=3–4 mice per genotype. (f) CXCR4 inhibition with AMD3100 effect in B16 colonization to the lungs of RERTFAKWTand RERTFAKKOmice. Bar chart shows fold change relative to PBS of mean number of B16 cells per lung area.n=10–16 mice per test. Scale bar, (a,c) 500 μm. NS, not statistically significant; *P<0.05; ***P<0.001, Student’st-test. Figure 7: Gr1 cells govern tumour cell colonization in RERTFAK KO mice. B16 tumour cells, previously labelled with red cell tracker CMTPX, were injected via the tail vein into RERTFAK WT , RERTFAK KO , BMFAK WT and BMFAK KO mice. ( a ) Lungs were harvested 2–5 h and 48 h after tumour cell injection to measure the numbers of tumour cells homing and colonizing in the lungs, respectively. Representative stereomicroscopic images of lung surfaces from RERTFAK WT and RERTFAK KO mice are given. ( b ) Bar charts represent mean number of B16 cells mm −2 lung section+s.e.m., n =5 mice per genotype. ( c ) Gr1 antibody-depletion of Gr1+ cells or CXCR4 inhibition with AMD3100 in RERTFAK WT and RERTFAK KO mice. Nonspecific IgG or PBS were used as a control. Mice were then injected with red cell tracker CMTPX labelled B16 cells. Representative stereomicroscope images of fresh lungs from both genotypes are given. ( d ) Bar chart shows fold change relative to IgG of mean number of B16 cells per lung area. n =10–12 mice per test. ( e ) Single-cell suspensions of blood from RERTFAK WT and RERTFAK KO mice 2 h post tumour cell injection via the tail vein were analysed by flow cytometry. Bar charts show numbers of CD45 + CD11b + Gr1 hi Ly6C lo (PMN) in blood. n =3–4 mice per genotype. ( f ) CXCR4 inhibition with AMD3100 effect in B16 colonization to the lungs of RERTFAK WT and RERTFAK KO mice. Bar chart shows fold change relative to PBS of mean number of B16 cells per lung area. n =10–16 mice per test. Scale bar, ( a , c ) 500 μm. NS, not statistically significant; * P <0.05; *** P <0.001, Student’s t -test. Full size image To examine the direct requirement of Gr1 + cells in tumour cell colonization, RERTFAK WT and RERTFAK KO mice were given two doses of a Gr1-blocking antibody (RB6-8C5), to deplete Gr1 + cells one day before and on the day of B16 melanoma cell injection via the tail vein. An isotype-matched antibody was used as a negative control. Efficient depletion of Gr1 + cells was confirmed at 2–5 and 48 h post tumour cell injection ( Supplementary Fig. 10B ). The control antibody treatment had no effect on the increased colonization observed previously in RERTFAK KO mice when compared with RERTFAK WT controls. Gr1 + cell depletion had small effect in RERTFAK WT animals but, however, had decreased tumour cell colonization in RERTFAK KO mice ( Fig. 7c,d ). These data suggest that the elevated number of Gr1 + cells in mice lacking stromal FAK is a critical regulator of the elevated tumour metastasis observed. In addition, RERTFAK WT and RERTFAK KO mice were given a Cxcr4 inhibitor AMD3100 or phosphate-buffered saline (PBS) as a control on the day of B16 melanoma cell injection via the tail vein. Cxcr4 inhibition was sufficient to decrease blood granulocyte levels soon after tumour cell injection ( Fig. 7e ). Importantly Cxcr4 inhibition had no effect in RERTFAK WT but decreased RERTFAK KO tumour cell colonization ( Fig. 7c,f ). Together these data suggest that Gr1 cell numbers and Cxcr4 signalling are important drivers for the increased tumour cell colonization observed in the absence of stromal FAK. Here we show that loss of FAK in the haematopoietic compartment is sufficient to augment metastasis. This is unexpected and highlights a mechanism by which metastasis is regulated. The overexpression of FAK in cancer cells, combined with it essential role in cell migration, has implicated this molecule as a positive regulator of cancer progression [5] , [54] , [55] . High levels of both FAK and Src can be indicative of poor prognosis and tumour recurrence in a variety of cancers [5] and these data have been interpreted to suggest that inhibitors of FAK may control cancer growth and progression. Indeed several reports have shown that inhibition of FAK, often in combination with the inhibition of other targets, can suppress tumour growth and metastasis [9] , [10] , [11] . In contrast, possible negative roles for FAK in tumour progression have also been reported [12] , [13] . For example, FAK expression is not a prognostic marker for colon adenocarcinoma patients and FAK expression does not correlate with survival [56] ; loss of tumour FAK is actually associated with increased metastasis in cervical cancer [12] ; pharmacological inhibition of Src can suppress metastasis without affecting FAK activation [57] ; and under some oncogenic conditions, such as those initiated by Ras, metastasis is promoted by dephosphorylating FAK [13] . Although various mechanisms have been discussed to explain how tumour cell FAK might control metastasis, what was not known was whether the absence of FAK in the stromal, and especially in the haematopoietic compartment, has any impact on metastasis. In contrast to previous data examining the tumour cell compartment, using a genetic ablation approach our data show that loss of stromal, and in particular, haematopoietic FAK is sufficient to actually enhance tumour metastasis. This implies that we may need to change our concept of FAK to reflect its potentially counteractive and pleiotropic roles during metastasis. In addition, although haematopoietic FAK deficiency was sufficient to increase metastatic burden, it did not affect primary tumour size or invasiveness suggesting that this initial step of tumorigenesis is not dependent on haematopoietic FAK. Furthermore, our data also show that genetic ablation of FAK in both the stromal and cancer compartments simultaneously also results in enhanced metastasis suggesting that loss of FAK globally is not sufficient to reduce metastasis. Our data imply that haematopoietic FAK acts as a negative regulator of metastatic dissemination and raise the question of which cells are responsible for this phenotype. Haematopoietic homeostasis is dependent on HSCs that have the ability to self renew and maintain lineage differentiation potential [58] , [59] and it has been hypothesized that disrupting interactions between HSCs and bone marrow stroma affects HSC fate [60] , [61] , [62] . Here, we observed that the absence of stromal FAK induced an increase in numbers of LT-HSCs and CMP within the bone marrow. Importantly FAK KO HSCs present higher levels of the transcription factor PU.1 and lower levels of GATA-1 —both hallmarks of commitment to a myeloid lineage [44] , [45] , [46] , [47] . Interestingly FAK has been shown to regulate other GATA family transcription factors [63] . This shift towards myeloid lineage commitment did not correlate with compensation within the bone marrow by Pyk2, or other focal contact proteins such as vinculin, paxillin or talin. Instead, our data established that loss of haematopoietic FAK can deregulate the HSC niche, an observation that is supported by recently published work demonstrating that FAK is preferentially expressed in HSCs and that loss of bone marrow FAK in Mx1-Cre;FAKfl/fl mice induced an increase in activated HSCs [42] . More importantly, our present data identifies a role for haematopoietic FAK in controlling myeloid lineage commitment programme and raised the question of whether this could be the main driver of the tumour metastasis observed. The changes in haematopoietic homeostasis that resulted in increased CMP levels were reflected in the periphery by increased mobilization of granulocytes into the circulation as described before [48] , [49] . Increased numbers of granulocytic and monocytic CD11b + Gr1 + cells were observed in the blood and spleen of tumour-initiated RERTFAK KO mice when compared with controls. Overall our findings establish that haematopoietic FAK is important for the regulation of circulating myeloid cell numbers, which have been shown to correlate with metastasis burden [19] , [20] . Cell changes were also accompanied by significant increases in CXCL12 and C5/C5a in the serum of RERTFAK KO mice, known pro-metastatic cytokines that correlate with poor prognosis [50] , [53] . Increase in CXCL12 serum levels have been observed in GATA-1 low mice, a phenotype consistent with the low GATA-1 levels observed in FAK KO HSCs [64] . On the other hand, CXCL12 serum increase was accompanied by elevated levels of its receptor CXCR4 in FAK KO PMNs sorted from lung after tumour cell injection. CXCR4 is a granulocyte homing receptor so this suggests that stromal FAK deficiency induced not only a change in PMN numbers, but also in their function. The high levels of CXCR4 in FAK KO PMNs likely increase their propensity to respond to CXCL12 and home to sites of metastasis. Indeed, this has been shown to be one of the mechanisms that governs granulocyte infiltration to drive metastasis [50] , [51] . Interestingly C5/C5a has also been demonstrated to induce granulocyte recruitment in inflammatory conditions [65] . Conversely, analysis of lymphoid numbers within the lung at early time points after tumour cell injection showed a decrease in CD8 and CD4 T cells with no alterations in NK cell numbers in RERTFAK KO and BMFAK KO mice when compared with respective controls. Since no changes were observed in bone marrow common lymphoid progenitors, this suggested that, in contrast to myeloid cells, the recruitment of T cells to the lung was impaired. Granulocytic and monocytic CD11b + Gr1 + cells are also referred to as MDSCs. MDSCs are characterized by their ability to suppress CD8 and CD4 T cell proliferation and cytotoxicity and suppress NK cell activity, which, together, are thought to enhance metastasis [23] , [24] . Moreover C5/C5a has been shown not only to increase the infiltration of MDSCs, but also their immune suppressive properties, resulting in decreased infiltration of CD8 T cells in tumours [66] . Our data corroborated these findings and point towards a role for haematopoietic FAK deficiency in increasing not only numbers, but also recruitment of granulocytes to metastatic sites, thus generating a pro-metastatic microenvironment [27] , [28] , [29] . In fact depleting Gr1 + cells or inhibition of CXCR4 in RERTFAK WT and RERTFAK KO mice before tumour cell injection was sufficient to reduce tumour cell colonization in the lungs of RERTFAK KO mice to levels observed in RERTFAK WT control mice. Thus our work shows that loss of stromal FAK, via the upregulation of Gr1 + cell numbers and CXCR4 signalling, induces a permissive microenvironment at metastatic sites that facilitates the increased colonization by tumour cells observed in RERTFAK KO and BMFAK KO mice. These data suggest that the myeloid commitment and recruitment of these cells to metastatic sites in RERTFAK KO mice are a major driver of the elevated tumour cell colonization observed. In short, our findings establish a critical mean by which FAK regulates metastasis. Decreasing FAK levels in the stromal and haematopoietic compartment generates a pro-metastatic microenvironment that increases tumour metastasis. Given the importance of understanding the biology behind cancer metastasis, the impact of our study lies in unfolding a mechanism by which FAK in the stromal compartment regulates metastasis. Mice FAK fl/fl mice [30] were bred with RERTn ERT/ERT Cre [31] , [32] mice provided by Mariano Barbacid to generate FAK fl/fl mice that express CreERT2 under the control of the large unit of RNA polymerase 2 ( RERTn ERT/ERT Cre;FAK fl/fl ) on a mixed C57BL6/129 background. RERTn ERT/ERT Cre;FAK fl/fl and control FAK fl/fl mice were bred with RIP-Tag2 mice [33] provided by Douglas Hanahan generating RIP-Tag2;RERTn ERT/ERT Cre;FAK fl/fl and RIP-Tag2;FAK fl/fl mice, respectively. WT mice were maintained on a mixed C57/Bl6J/129 background, whereas RIP-Tag2 mice used for transplantation experiments were maintained on a C57/Bl6J background in standard ventilated cages in accordance with CR-UK and QMUL institutional and Home Office guidelines. Male mice were used as bone marrow donors. All experiments were approved by the Animal Research Ethics and United Kingdom Coordination Committee on Cancer Research guidelines and Home Office Regulations. RIP-Tag2 model RIP-Tag2;RERTn ERT/ERT Cre;FAK fl/fl and RIP-Tag2;FAK fl/fl mice were induced with daily tamoxifen in the chow (Harlan) at 8–9 weeks of age and were culled at 15 weeks of age. Lethally irradiated RIP-Tag2 mice were transplanted with bone marrow cells from male RERTn ERT/ERT Cre;FAK fl/fl or FAK fl/fl control mice at 6 weeks of age. Mice were induced with tamoxifen treatment in the chow at 8–9 weeks of age and were culled at 16 weeks of age. At necropsy, pancreas with peri-pancreatic lymph nodes, liver and lungs were fixed in 4% formaldehyde in PBS for subsequent immunohistochemical analysis. Invasion grading and metastasis analysis were performed by staining for Tag as described previously [35] . Paraffin-embedded sections of pancreas, liver and lungs were permeabilized in citrate buffer, blocked in 5% normal goat serum, incubated with rabbit anti-mouse large T cell antigen (Santa Cruz Biotechnology) antibody (1:200 dilution) overnight at 4 °C and anti-rabbit biotinylated secondary antibody (1:200 dilution) for 45 min at RT. ABC reagents (Vector Labs) were added and staining developed with DAB (Vector Labs) and couterstained with haematoxylin (Sigma-Aldrich). Five step-wise sections, 100 μm apart were analysed per tissue for all mice. Experimental metastasis assays RERTn ERT/ERT Cre;FAK fl/fl or RERTn ERT/ERT Cre control mice were given 3 mg of tamoxifen (Sigma-Aldrich) by gavage for 5 consecutive days and then daily tamoxifen in the chow until the end point of the experiment. Bone marrow transplanted mice were treated with tamoxifen starting 2–3 weeks post transplant. After 5–7 days of tamoxifen treatment, 0.5 × 10 6 tumour cells (B16F0 or B16F10—ATCC, mycoplasma free) resuspended in 100 μl of PBS were injected via the tail vein. Mice were examined for metastases at necropsy. Tissues were either fixed in 4% formaldehyde in PBS or snap-frozen in isopentane cooled in liquid nitrogen for subsequent immunohistochemical analysis. Bone marrow transplantation Female mice of at least 6–12 weeks of age were γ-irradiated with 2 × 500 rad doses, 3 h apart, to ablate the endogenous bone marrow. They were immediately rescued by tail vein injection of 1 × 10 6 freshly isolated bone marrow cells from male RERTn ERT/ERT Cre;FAK fl/fl or RERTn ERT/ERT Cre control mice resuspended in 0.1 ml sterile PBS. The mice were treated with enrofloxacin (Baytril, Bayer) until 2 weeks after bone marrow transplantation. RIP-Tag2 mice were transplanted at 6 weeks of age. Flow cytometry At different time points, mice were killed and cells isolated from bone marrow, blood, lungs and spleen, and cell surface phenotypes were determined by direct immunofluorescence staining with conjugated antibodies for mouse haematopoietic lineage-efluor450 and the anti-mouse antibodies CD117 (c-Kit)-APC, CD135 (Flt3)-PE, CD34-PE, CD16/32-PE-Cy7, CD45-efluor450, Gr1-FITC, Ly6C-APC and CD11b-PE (eBiosciences) and Ly6-A/E (Sca-1)-PerCP-Cy5.5 antibodies (Biolegend) all used at 1:100 dilution. Data were collected and analysed using the BD LSRII and FlowJo softwares. HSC isolation HSCs were isolated from lineage depleted or c-Kit-enriched bone marrow as described in refs 67 , 68 , using Miltenyi magnetic columns separation kits. The cells obtained were then stained with streptavidin PE-Cy7 (Biolegend) (lineage depleted cells) or lineage cocktail antibodies (BD Pharmingen) followed by streptavidin PE-Cy7 (c-Kit-enriched cells) plus anti-mouse c-kit-APC and Ly6-A/E (Sca-1)-Pacific Blue antibodies (Biolegend). Subsequently, Sca1 + c-Kit + Lin − (HSC) cells were isolated using a fluorescence-activated cell sorting Aria (Becton Dickinson, Franklin Lakes, NJ). Lung PMN isolation Single-cell suspensions of lung were obtained by mincing tissue and digesting in HBSS (without Ca, Mg) plus collagenase IV (2 mg ml −1 ) (Gibco) for 20 min at 37 °C, followed by 5 mM EDTA to stop the reaction and forcing through a 70-μm cell strainer. After lysing the red blood cells and washing in PBS with 2% fetal bovine serum, cells were blocked with Fc block (BD Pharmingen) for 15 min at 4 °C followed by incubation with the following antibody mix: CD45-efluor450, Gr1-FITC, Ly6C-APC and CD11b-PE (eBiosciences). Subsequently, CD45 + CD11b + Gr1 hi Ly6C lo (PMN) cells were isolated using a fluorescence-activated cell sorting Aria (Becton Dickinson). Gene expression analysis RNA was extracted from HSC and PMN using the RNeasy Micro Kit (Qiagen) and recommended protocol. cDNA syntesis was performed in 20–50 ng of RNA using the Sensiscript RT Kit (Qiagen) according to manufacturer’s instructions. For real time PCR each 20 μl reaction contained test cDNA (1–2 μl), 10 μl Platinum SYBR Green qPCR SuperMix-UDG with Rox (Invitrogen), 300 nM of each forward and reverse primer and nuclease free H 2 O in an individual well of a 96-well plate. The following primer sets were used per reaction: GAPDH fw (5′-CTGCACCACCAACTGCTTAG-3′) and GAPDH rev (5′-GTCTTCTGGGTGGCAGTGAT-3′); FAK fw (5′-AACAGCTATTTGATTTCTTCTCAAAGT-3′) and FAK rev (5′-TCTTTTGCTAGATGCTAGGTATCTGT-3′); PU.1 fw (5′-CGGATGACTTGGTTACTTACG-3′) and PU.1 rev (5′-GTAGGAAACCTGGTGACTGAG-3′) [69] ; Gata-1 fw (5′-ATTCCTGGGGGCTCACCTTATG-3′) and Gata-1 rev (5′-TCCACAGTTCACACACTCTCTGGC-3′) [69] ; CXCR4 fw (5′-TCCAACAAGGAACCCTGCTTC-3′) and CXCR4 rev (5′-TTGCCGACTATGCCAGTCAAG-3′). The following conditions were used to run the PCR amplification process: 50 °C for 2 mins, denaturation at 95 °C for 10 mins followed by 40 cycles at 95 °C for 15 s and 1 min annealing/extension at 60 °C. Data analyses were accomplished using the StepOne Plus Real Time PCR machine (Applied Biosystems). Data were normalized to endogenous GAPDH and fold changes in gene expression were calculated using the comparative CT method. Immunofluorescence For immunofluorescence staining for Gr1, 5 μm frozen lung sections were fixed in 100% acetone for 10 min, blocked in 5% normal goat serum (Sigma-Aldrich) for 1 h, incubated with rat anti-Gr1 (clone RB6-8C5—BD Pharmingen) primary antibody (1:50 dilution) overnight at 4 °C and anti-rat Alexa-Fluor-488 (Molecular Probes) secondary antibody (1:200 dilution) for 45 min at room temperature and finally mounted with Prolong anti-fade with 4',6-diamidino-2-phenylindole (DAPI; Molecular Probes). Gr1 + cell numbers were quantified microscopically in at least five different fields per section. Values are given relative to total number of cells as assessed by the DAPI signal. Cytokine analysis in serum At indicated time points mice were killed, blood collected by heart puncture, left to clot for 2 h at room temperature and centrifuged at 2,000 g for 20 min. Mouse cytokine arrays (Proteome Profiller ARY006—R&D Systems) were processed according to manufacturer’s instructions using 100 μl of serum per membrane. Pixel analysis was used for quantification using Image J software. In vivo homing/colonization assays B16F0 cells, previously labelled with red cell tracker CMTPX (Molecular probes, Invitrogen, Life Sciences), were resuspended at 0.5 × 10 6 cells per 100 μl of PBS and injected via the tail vein into mice. At 2 or 48 h post inoculation, mice were killed and lungs fixed in 4% paraformaldehyde. Lungs were dissected, photographed using a Leica MZ16F fluorescence stereomicroscope, snap-frozen in OCT (OCT Killik, Bio-Optica, IT) and 5 μm cryosections were prepared for analysis. Total numbers of red fluorescent tumour cells were quantified and normalized for the total number of DAPI-positive nuclei for each section using a Zeiss Axioplan microscope (Zeiss). Gr1 depletion experiments Mice were given 50 μg of rat anti-mouse Gr1 antibody (RB6-8C5, eBiosciences) or rat anti-mouse IgG2b κ isotype control antibody (eBiosciences) in 100 μl PBS one day before and on the day of tumour cell injection. Homing/colonization assays were performed as described in the In vivo homing/colonization assays section. CXCR4 inhibition experiments Mice were given 5 mg kg −1 of AMD3100 (Sigma) or PBS intraperitoneal on the day of tumour cell injection and following days until harvesting. Homing/colonization assays were performed as described in the In vivo homing/colonization assays section. At 48 h time point mice were harvested within 60–90 min after inhibitor treatment. Statistical analysis Results are presented as means±standard error of the mean (s.e.m.) for at least 2–3 independent experiments, unless otherwise stated. The sample sizes used were based on level of changes and consistency expected. Statistical significance was reported as appropriate. Experimental metastasis and RIP-Tag2 data analysis of statistical significance was performed using nonparametric Mann–Whitney and χ 2 tests. All other data sets were analysed for statistical significance using Student’s t -test. For both tests P <0.05 was considered statistically significant. Sample sizes were chosen on the basis of the level of changes expected. No randomization methods were used. During animal experiments, the investigator was blinded to the genotype of the animals under study. How to cite this article: Batista, S. et al. Haematopoietic focal adhesion kinase deficiency alters hematopoietic homeostasis to drive tumour metastasis. Nat. Commun. 5:5054 doi: 10.1038/ncomms6054 (2014).